A hydrothermal anvil made of graphene nanobubbles on diamond The hardness and virtual incompressibility of diamond allow it to be used in high-pressure anvil cell. Here we report a new way to generate static pressure by encapsulating single-crystal diamond with graphene membrane, the latter is well known for its superior nano-indentation strength and in-plane rigidity. Heating the diamond–graphene interface to the reconstruction temperature of diamond (~1,275 K) produces a high density of graphene nanobubbles that can trap water. At high temperature, chemical bonding between graphene and diamond is robust enough to allow the hybrid interface to act as a hydrothermal anvil cell due to the impermeability of graphene. Superheated water trapped within the pressurized graphene nanobubbles is observed to etch the diamond surface to produce a high density of square-shaped voids. The molecular structure of superheated water trapped in the bubble is probed using vibrational spectroscopy and dynamic changes in the hydrogen-bonding environment are observed. Graphene is commonly thought of as a two-dimensional carbon flatland. This ideal picture, however, is valid only in special cases like suspended graphene [1] , [2] , [3] , graphene grown epitaxially on SiC [4] or supported on low-surface energy substrate like hexagonal boron nitride [5] , [6] . In fact, monolayer graphene is inclined towards deformation in the third dimension because of its large ratio of in-plane rigidity to bending rigidity. In most cases, the substrate supporting graphene induces buckling under compression and creates ripples and blisters, which sets a limit on the mobility of its charge carriers due to flexural phonons. A recent study by Pan et al [7] observed sub-micron bubbles due to the biaxial compressive strain in the graphene/hexagonal boron nitride heterostructure after thermal cycling. Compressive strain between the lattice-mismatched Ru and graphene creates a buckling instability, which manifests as periodic blistering (Moire humps) on the sheet [8] , [9] ; these blisters can be sintered to produce geometrically shaped bubbles on the metal [10] , giving rise to electrodynamics that are coupled to the strain texture. Although the strain properties of the bubbles have been studied using spectroscopic methods, the physical properties of trapped species inside the bubble have not been investigated. One interesting possibility, which has not been considered thus far, is the reactivity of the trapped fluid in the impermeable graphene bubble. The ability of graphene to seal the interface between itself and the supporting platform ensures the mechanical stability of these bubbles and provides a unique anvil cell for probing the dynamics of fluids trapped within this impermeable membrane, at conditions beyond the critical point of the fluid. In almost all reported cases to date, the occurrence of the bubbles is sporadic over the graphene surface [11] , [12] . To record sufficient signal strength when probing the molecular structure of water trapped within each bubble, a high areal density of nanobubbles is needed. The diamond–graphene interface is selected to meet this requirement. First, the lattice mismatch between diamond and graphene will produce interfacial stress, which induces periodic rippling on graphene. Second, covalent bonding between the two phases can occur when the surface of diamond is reconstructed thermally. Although the phases of diamond and graphite are known to coexist in surface-graphitized nanodiamond particles or during the initial nucleation stages of diamond growth [13] , [14] , [15] , [16] , there is no clear insight into how graphene interfaces with diamond both structurally and electronically. The metallic-sp 2 and dielectric-sp 3 interface offers the perfect environment for studying the complex interplay between electronic and lattice degrees of freedom for the creation of new functionalities. Here we transfer a chemical vapour deposited (CVD)-grown graphene monolayer onto single-crystal diamond (100) and thermally anneal the interface to the reconstruction temperature of diamond to study the morphological evolution at the interface. We show that interfacial bonding results in the growth of high-density nanobubbles across the graphene sheet. The resultant nanobubble ‘mat’ has a distinct topographical and electronic landscape. Most interestingly, each graphene nanobubble (GNB) that interfaces with diamond acts as a hydrothermal anvil cell: the water entrapped is transformed into compressed, hot water (supercritical) that is highly corrosive to even one of the hardest known materials, diamond. GNBs on diamond A consequence of graphene being a soft membrane is that it can be strain-engineered to become highly corrugated by modifying its adhesion to the substrate. A CVD-grown graphene monolayer sheet was transferred onto a diamond (100) crystal. After annealing the graphene–diamond interface at 1,275 K for 45 min in ultrahigh vacuum, GNBs with a density of ~8 × 10 10 cm −2 ( Fig. 1 ) appear. Each GNB measures about ~2 nm in height and has diameters that range from 5 to 30 nm ( Fig. 1c ). The annealing temperature of 1,275 K causes the dehydrogenation of the hydrogen-terminated diamond (100). Dangling bonds, which are created during dehydrogenation, bond instantaneously with graphene sheet, and the non-bonded part of the graphene sheet buckles to relieve the compressive stress arising from the interfacial bonding. This reconstruction process happens spontaneously once the interface is activated thermally, as can be seen from the molecular dynamic (MD) simulations presented later (Fig. 4). We have carried out control studies on mechanically exfoliated graphene and found that GNBs of similar size and density can be generated for wet-transferred exfoliated graphene sheet on diamond, thus the bubble formation is not specifically influenced by the grain boundaries because the sizes of crystalline domains are expected to be quite different in CVD and exfoliated graphene ( Supplementary Fig. S1 ). Valence band spectroscopy in Fig. 2a revealed that the intensity of the characteristic p orbital peak in graphene was reduced with the formation of GNBs; we deduce that this is due to partial re-hybridization of its molecular orbitals following interfacial bonding with diamond. 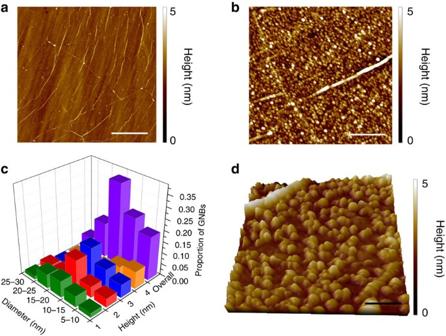Figure 1: AFM images of GNBs. (a) Topography of G on diamond after transfer. (b) Topography of GNBs on diamond. Scale bar, 500 nm (aandb). (c) Histogram of the diameter and height distribution of GNBs and (d) High-resolution three-dimensional topography representation of GNBs on diamond. Scale bar, 100 nm. Figure 1: AFM images of GNBs. ( a ) Topography of G on diamond after transfer. ( b ) Topography of GNBs on diamond. Scale bar, 500 nm ( a and b ). ( c ) Histogram of the diameter and height distribution of GNBs and ( d ) High-resolution three-dimensional topography representation of GNBs on diamond. Scale bar, 100 nm. 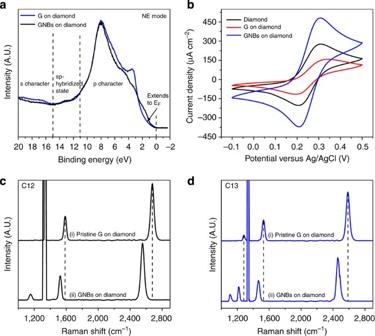Figure 2: Probing the electronic structure and properties before and after the formation of GNBs. (a) Valence bands of flat G and GNB on diamond. (b) Electrochemical cyclic voltammetry of diamond, graphene-on-diamond and GNBs-on-diamond using 1.0 mM Fe(CN)63−/4−in 1 M KCl. (c) C12 Raman spectra of (i) flat graphene-on-diamond before GNB formation, (ii) GNBs on diamond and (d) C13 Raman spectra of (i) flat graphene-on-diamond before GNB formation and (ii) GNBs on diamond. Full size image Figure 2: Probing the electronic structure and properties before and after the formation of GNBs. ( a ) Valence bands of flat G and GNB on diamond. ( b ) Electrochemical cyclic voltammetry of diamond, graphene-on-diamond and GNBs-on-diamond using 1.0 mM Fe(CN) 6 3−/4− in 1 M KCl. ( c ) C12 Raman spectra of (i) flat graphene-on-diamond before GNB formation, (ii) GNBs on diamond and ( d ) C13 Raman spectra of (i) flat graphene-on-diamond before GNB formation and (ii) GNBs on diamond. Full size image Strained GNBs Strain, which affects the phonon frequency and which depends on the anharmonicity of the interatomic potentials, can be studied using Raman spectroscopy [12] . Sp 2 -hybridized CVD graphene layer is characterized by its G, D and 2D (second-order D peak) peaks, which reside at 1,580, 1,360 and 2,680 cm −1 , respectively [17] . G peak corresponds to the doubly degenerated E 2g phonon at the Brillouin zone centre. The 2D peak originates from a scattering process where momentum conservation is obtained by the participation of two phonons with opposite wavevectors ( q and − q ). The D peak is usually selection-rule forbidden but is activated by lattice defects. Raman spectrum was recorded using a scanning atomic force microscope (AFM)-Raman probe so that the Raman features collected from a region that is covered densely by the GNB can be contrasted with another region where the graphene is relatively flat. Figure 2c shows that the Raman spectrum collected from the GNB-covered region is red-shifted as compared with spectrum recorded at the flat regions. This can be explained by the elongation of C–C bonds in the tensile strained GNB. In particular, the G-peak position decreases from 1,586 to 1,525 cm −1 , whereas the 2D band shifts from 2,678 to 2,553 cm −1 when moving from the flat to curved regions. The full-width at half-maximum of the 2D peak remains unchanged at about 30 cm −1 . These observations suggest that the lattice of graphene is biaxially strained [18] . Using d ω /dε , where ω is the Raman frequency and ε is the % strain applied to CVD graphene [19] , the Grüneisen parameter γ was calculated to be γ =1.30 using the equation [20] γ =−1/ ω o ( d ω / dε ), where ω o is the Raman frequency with no applied strain. The strain value experienced by GNBs is then calculated to be ~1.5%. However, the strain value probed by Raman spectroscopy here is underestimated because of the large laser spot size of the Raman probe relative to individual nanobubbles. Alternatively, the strain quantification of each individual GNB can be judged from its physical parameters. Because σ = pr 2 /2 th , strain is related to stress by ε =(1− ν 2 )/ E ) σ , where σ is the stress experienced at the apex of the graphene bubble, P is the differential pressure across the membrane responsible for the magnitude of deflection, r is the radius of the GNB, t is the thickness of graphene and h is the height of GNB. Using AFM to determine the mean r and h of the bubbles, ε was estimated to be ~6% for the GNB. Besides the commonly observed G and 2D bands in pristine graphene, an unusual peak residing at ~1,150 cm −1 is observed to emerge upon the formation of GNBs ( Fig. 2c ). This peak is often recognized as the fingerprint band of nanocrystalline diamond crystals. Ferrari et al [21] assigned it to mixed sp 3 − sp 2 bonded phases and trans-polyacetylene groups present on the surface and grain boundaries of nanocrystalline diamond. One possibility is the bonding of diamond to graphene breaks the honeycomb sheet into mixed sp 3 − sp 2 bonded phases, and trans-polyacetylene domains appear on the modified graphene, which is bonded to diamond. At the same time, a widening of the full-width at half-maximum of the 1,332 cm −1 peak ( Fig. 2c ) is observed with the growth of GNBs, and this can be attributed to the increased density of defects following interfacial bonding. To avoid the overlap between the defect peak of graphene and the first-order phonon peak of single-crystal diamond (situated at 1,332 cm −1 ), the Raman spectrum of C13-enriched graphene was recorded. The D peak of graphene, which is defect-related, is observed to increase with the formation of GNBs ( Fig. 2d ) and similar downshifting of the G and 2D peaks is also observed for the curved regions of the GNBs. Unique properites of GNBs Pristine graphene shows excellent in-plane electrical conductivity. However, because of the anisotropic nature of its electron delocalization, it is known to be electrochemically sluggish for charge transfer in the direction normal to its basal plane [22] . An exception is found, however, in the case of GNB, because its strained surfaces means that the flat-lying 2 p orbitals are distorted, and midgap states will be created to which enhanced charge transfer can occur. The curvature in GNB also causes an asymmetric distribution of π electrons outside and inside graphene sheet [23] , bestowing greater electrochemical reactivity on its exterior. Cyclic voltammetry of Fe(CN) 6 3−/4− redox couple was selected to examine the heterogenous charge-transfer mechanism before and after the formation of GNBs. In this case, the graphene sheet is transferred to a conducting, boron-doped diamond crystal. Using an inner sphere redox couple, which is sensitive to both the density of electronic states and surface microstructure, charge-transfer kinetics can be calculated from the peak-to-peak separation in the voltammograms ( Fig. 2b ). The results show that the charge-transfer rate follows the order of: GNBs on diamond>diamond>flat G on diamond, as summarized in Table 1 . The cathodic and anodic currents of GNBs on boron-doped diamond electrode ( Supplementary Fig. S2 ) show a linear relationship with the square root of the scan rated ranging from 25 to 125 mV s −1 , which is in good agreement with the Randles Sevcik equation describing reversible reactions controlled by semi-infinite linear diffusion. Boron-doped diamond is known to be a good electrode for electrochemistry, but what is striking here is the enhanced electrochemical response when its surface is modified by GNBs. Table 1 Calculated apparent heterogeneous electron-transfer rate constants and capacitances. Full size table Insights into the formation of GNBs The GNB-on-diamond sample was introduced into a Fourier transform infrared spectroscopy (FTIR) in-situ cell evacuated to 1 × 10 −4 Torr. FTIR measurements reveal that residual water from the graphene-transfer process is trapped at the GNB–diamond interface because of the impermeability of graphene [24] ( Fig.3d ). Surface-physisorbed water typically desorbs readily in vacuum once the sample is heated slightly due to its weak adsorption energies on hydrophobic surface. However, we observed that the water-related OH vibrational bands persist up to the highest heating temperature in GNB-on-diamond (>773 K); this is possible only if the water molecules are trapped at the GNB–diamond interface. The observation of trapped water echoes a recent study that demonstrated the imaging of trapped water between two graphene membranes using high-resolution transmission electron microscopy [25] . It is worth mentioning that the impermeability of the graphene membrane to atoms and molecules has been predicted by Leenaerts et al [26] using first-principles density functional theory investigation. 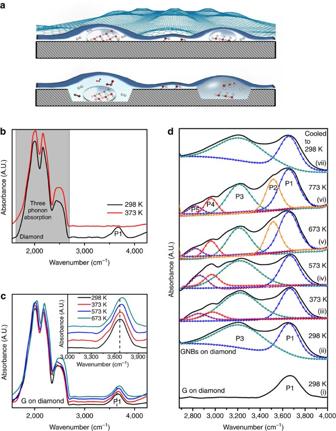Figure 3: Schematic diagram and vibrational spectroscopy of graphene and diamond. (a) Schematic representation showing water cluster in GNB and weakly interacted water molecules underneath flat G graphene on diamond (top panel). Etching of diamond by supercritical water (bottom panel). FTIR spectra showing OH-stretching peak of water measured on (b) diamond, where raising temperature to 373 K results in the desorption of water (c) Flat G on diamond showing peak at 3,650 cm−1due to the presence of trapped, weakly bonded water molecules; (d) (i) Flat G on diamond; (ii)–(vi) After formation of GNBs on diamond and heating the GNB at a range of temperatures and (vii) Cooling down to room temperature. Figure 3: Schematic diagram and vibrational spectroscopy of graphene and diamond. ( a ) Schematic representation showing water cluster in GNB and weakly interacted water molecules underneath flat G graphene on diamond (top panel). Etching of diamond by supercritical water (bottom panel). FTIR spectra showing OH-stretching peak of water measured on ( b ) diamond, where raising temperature to 373 K results in the desorption of water ( c ) Flat G on diamond showing peak at 3,650 cm −1 due to the presence of trapped, weakly bonded water molecules; ( d ) (i) Flat G on diamond; (ii)–(vi) After formation of GNBs on diamond and heating the GNB at a range of temperatures and (vii) Cooling down to room temperature. Full size image The OH stretch of water presents an extremely broad band between 3,000 and 3,700 cm −1 , which is usually described by the four state model [27] in terms of the strength of hydrogen bonding. The intra-molecular OH stretch is highly dependent on the hydrogen-bond coordination of the proton [28] . A strong hydrogen bonding results in a weakening of the OH oscillator, a red shift in energy and a broadening of the spectral peak. As shown in Fig. 3d , a relatively sharp peak labelled as P1 at ~3,650 cm −1 , which is characteristic of free OH bond of water molecules, is observed at the bare diamond surface but this peak vanishes upon slight heating, and only the intrinsic 3 phonon absorption peaks of diamond [29] ( Fig. 3b ) remain. Thus, we can conclude that physisorbed water desorbs completely from the surface at elevated temperatures. Peak P1 is also observed at diamond surface encapsulated by flat graphene sheet ( Fig. 3c ), but in this case, it survives even after high-temperature annealing, suggesting that the water is trapped at the graphene–diamond interface. The persistence of P1 as temperature increases suggests that a large body of water molecules adsorbing on hydrophobic surface have weak hydrogen-bonding interactions. For GNB–diamond, it is noteworthy that in addition to P1, a red-shifted broad band (P3) at ~3,220 cm −1 , which is characteristic of strong hydrogen bonding, is present at room temperature. P3 can be assigned to the condensation of water inside the bubbles. When the GNB–diamond sample is heated to increasingly higher temperature, another red-shifted P4 peak at 2,967 cm −1 emerges, which is indicative of increased clustering. At 673 K, the intensity of the 3,220 cm −1 peak is observed to weaken, and a blue shifted sharp peak P2 appears at 3,510 cm −1 . At this point, the weakening of the hydrogen bonding can be interpreted as the emergence of supercritical phase in some of the bubbles [30] , [31] , [32] . Previously, Tassaing et al [31] observed a broadening of vibrational bands, leading to a broad band with two maxima at about 3,650 and 3,550 cm −1 and a shoulder at 3,250 cm −1 as water approaches critical conditions. The critical temperature of water is 647 K, and the properties of water >674 K and at pressures higher than 2.21 MPa (critical pressure) differ significantly from those of ambient water. Supercritical water has a density between that of water vapour and liquid at standard conditions, reduced intermolecular bonding and exhibits high gas-like diffusion rates along with high liquid-like collision rates. A significantly reduced dielectric constant [33] (~20) allows it to act as an aggressive solvent for organic material. From the infrared spectra, it can be inferred that the trapped water molecules are rather inhomogeneous in its bonding environment; some water molecules trapped in the bubble undergoes clustering as pressure (temperature) increases, as reflected from increasingly stronger hydrogen-bonding environment (P4 and P5), whereas other water molecules, possibly trapped under flat part of the graphene sheet, do not cluster, as judged from the persistence of peak P1. It must be pointed out that peaks P2, P4 and P5 are dynamic features that are observed only at high temperatures; they decrease in intensities once the sample is cooled to room temperature ( Fig. 3d (vii) ). GNBs as high-pressure reactors for etching of diamond After heating the GNB–diamond sample over 1 h at 1,375 K, numerous nanometer-sized square voids appear on the diamond surface with a density of 9 × 10 9 cm −2 . 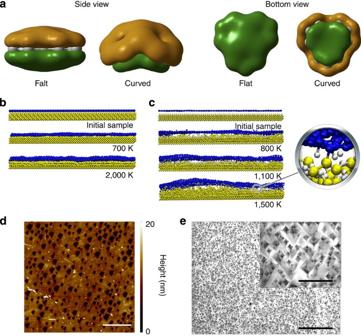Figure 4: GNB formation, growth and void generation on diamond. (a) Density functional theory simulation of ground electronic states of flat and curved graphene at B3LYP/6-31 G* level. (b,c) MD simulation of the buckling of graphene on diamond (b) Graphene on C(100)−(2 × 1). (c) Graphene on dihydride-terminated diamond (denoted as 2 H C(100)−(2 × 1), where bubble formation can be seen after heating. (d) AFM topography image of voids generated on diamond and (e) Scanning electron microscope image of etched diamond, inset is image zoomed in by 20 times. Scale bar, 0.3, 1 and 0.05 μm (d,eand inset ofe, respectively). Figure 4e shows the scanning electron microscope image of these nanovoids, which have an average width of ~40 nm The square etched pits follow the crystallographic expectation of the 100-faceted diamond. The occurrence of etched pits is intriguing as vigorous chemical or physical treatments, in the presence of transition metal catalysts, are usually needed to etch diamond. Control studies where the diamond crystal was heated alone in air or in vacuum at the same temperature failed to reproduce the etched pits that were observed when the diamond crystal was encapsulated by graphene membrane. At elevated temperatures, GNBs can be transformed into a hydrothermal reactor because of its impermeability [21] , [34] . Trapped water molecules inside can be transformed into supercritical fluid, which is highly corrosive to organic medium. For example, supercritical water has been used in the oxidation of methane to produce CO and CO 2 at 25 MPa and temperature >773 K [35] . Figure 4: GNB formation, growth and void generation on diamond. ( a ) Density functional theory simulation of ground electronic states of flat and curved graphene at B3LYP/6-31 G* level. ( b , c ) MD simulation of the buckling of graphene on diamond ( b ) Graphene on C(100)−(2 × 1). ( c ) Graphene on dihydride-terminated diamond (denoted as 2 H C(100)−(2 × 1), where bubble formation can be seen after heating. ( d ) AFM topography image of voids generated on diamond and ( e ) Scanning electron microscope image of etched diamond, inset is image zoomed in by 20 times. Scale bar, 0.3, 1 and 0.05 μm ( d , e and inset of e , respectively). Full size image The pressure inside a GNB can be estimated from its deformation from a flat membrane using Hencky’s solution for the geometrically nonlinear response of an isotropic elastic membrane subjected to a pressure difference Δ p across the membrane. This solution provides the membrane profile in the form of an infinite series in radial position, and also the relationship between the pressure difference and bubble height, Δ p = K ( ν ) ( Eth 3 )/ r 4 . Here E is the Young’s modulus, ν is Poisson ratio, t is the membrane thickness, r is the radius of the bubble and K ( ν ) is the coefficient that is dependent on the Poisson ratio. For graphene, we take ν =0.16, and so K( ν =0.16)=3.09 (ref. 36 ). The mean h and r values derived from AFM imaging are employed for estimation of pressure difference across a typical GNB. The pressure that is built up in a typical GNB of 2 nm in height and 10 nm in radius is calculated to be approximately 1 GPa. Alternatively, by considering a monolayer of water adsorbed on the surface of diamond and trapped within the GNB, the pressure estimated in the bubble using ideal gas law also arrived at a value of ca. 1 GPa. This value obtained lies within the pressure–temperature regime where etching of diamond is possible [37] . The etching of diamond octahedrons at 1,375 K and 10 9 Pa has been previously reported with water and oxygen acting as etchants [37] , [38] . Inside the bubbles, the superheated water is known to have enhanced solubility for non-polar organic materials. It is interesting to reflect on the chemical robustness of the GNB relative to the diamond that is encapsulating. Figure 4a shows the p z orbital isosurface wavefunction (isoval=0.02 A.U.) of flat and curved graphene calculated using density functional theory (at B3LYP/6-31G*). In contrast to the evenly distributed electronic density of a flat graphene plane, the curvature in GNB produces an asymmetric distribution of π electrons on its outer and inner surface. Outward rotation of orbitals enhances local density of states and bestows higher reactivity on the outer surface of the GNB. In contrast, orbitals at the inner surface of the GNB ( Fig. 4a ) are rotated inwards to result in a diminished electron cloud, thus resulting in reduced reactivity of concaved graphene surface [39] . With increasing temperature, the GNB bursts finally, and remnants of the torn graphene sheets can be observed using AFM imaging ( Fig. 4d ). Raman spectroscopy of the surface at this point reveals poly-acetylene-like fragments on the pit-covered diamond ( Supplementary Fig. S3 ). To obtain an atomistic insight into the formation mechanism of GNBs on diamond, we carried out classical MD simulations using reactive empirical bond-order potential [40] , [41] and reactive force field [42] . Diamond (100) slab with an atom density of 1.56 × 10 15 cm −2 atoms and a size of 35 × 35 × 0.45 nm 2 was built by six layers of atoms, each containing 20 000 atoms. Graphene (C(0001) sheet with a surface atom density of 3.65 × 10 15 atoms cm −2 and containing 48 720 atoms was placed Z =2.5 Å away from the surface of diamond to ensure that graphene and diamond are not covalently bonded at first. We first test the possibility of bonding interactions between graphene and a bare diamond surface. The bare diamond surface is a reconstructed (100)−(2 × 1) surface truncated by dimer row formation. No interfacial bonding between diamond and graphene is observed when the system is heated to 700 K, and only a minor rippling of graphene is observed (see Fig. 4b at 700 K). The reason of the rippling is the lattice mismatch between diamond (100) and graphene. The amplitude of rippling increases with the heating temperature; however, even at 2000 K, the height of the ripples does not exceed 5 Å ( Fig. 4b at 2,000 K). A different situation exists when a dihydride-terminated (denoted as 2H: C(100)−(2 × 1)) diamond surface interacts with graphene ( Fig. 4c ). Upon desorption of hydrogen atoms at 1,100 K, our MD simulation shows clearly that graphene–diamond bonding occurs instantaneously ( Fig. 4c ). The graphene–diamond bonding produces ripples on graphene sheet. At ≥1,500 K, part of graphene sheet erupts into bubbles ( Fig. 4c at 1,500 K) due to pressure created by desorbing hydrogen molecules. At even higher temperature, breakage of interfacial C–C bonds between graphene and diamond resulted in the delamination of GNB from diamond surface. These simulations confirm that the formation of GNB on the diamond surface is initiated by the interfacial bonding between diamond and graphene. Interfacial bonding seals the edges and prevents the graphene sheet from delaminating from diamond, thus desorbed gaseous species are trapped effectively within the bubbles. Gasification of surface-adsorbed species like hydrogen and water create pressure inside the bubble because of impermeability of graphene membrane. It can be appreciated that the size of the bubble will scale with the amount of trapped water molecules, which is confirmed by our experiments on oxygenated diamond surfaces, which are hydrophilic and trapped a greater volume of water ( Supplementary Fig. S4 , Supplementary Table S1 and Supplementary Note 1 ). The ability of graphene to undergo out-of-plane bonding with diamond is essential for sealing the edges of the bubble, otherwise on non-bonding substrate, a decohesion of the graphene membrane occurs and no bubble formation occurs (refer to Supplementary Fig. S4 ). The technological implication of the present work extends to supercritical fluid-assisted etching of solid surfaces, as well as fabricating new types of high-pressure anvil cell using graphene membrane. Because of the transparency and high thermal conductivity of graphene, it can serve as an optical window for laser-assisted etching where exponential increase in etch rates can be brought about by the synergistic effects of photoexcitation and ultrahigh pressure. Finally, the encapsulation of fluids between graphene bubbles and diamond allow supercritical fluids to be probed spectroscopically using a wide range of radiation ranging from X-ray, infrared light to gamma rays. In conclusion, the graphene–diamond interface undergoes bonding at high temperature to transform the graphene layer on top of the diamond into an undulating sheet of nanobubbles. There are several important outcomes. First, the GNBs-coated diamond surface shows enhanced electrochemical activity compared with the surface encapsulated by a flat graphene sheet, due to the highly strained structure of the former. Second, the GNBs can trap fluid within and act as hydrothermal anvil cells when the diamond–graphene interface is heated to high temperatures. Interestingly, we discover that superheated water trapped inside the nanobubbles is highly corrosive and etches diamond. This work shows the first example of using an impermeable atomic membrane for trapping fluid at supercritical conditions, where the hydrogen-bonding dynamics of water molecules at high temperature and pressure can be studied using in situ FTIR. Thus, the graphene–diamond hydrothermal anvil can serve as a useful bench-top construct for investigating the dynamic chemistry of supercritical phases in fluids. CVD growth and transfer of graphene The graphene sheets used in this study were grown by CVD following previous reported procedures [43] . The process was carried out in a quartz tube at reduced pressure with copper as a catalyst for G growth. The copper foil (thickness of 25 μm, purity of 99.8%) was heated at 1,275 K under a 10-sccm flow of H 2 (~400 mTorr) to reduce the oxide present, increase the grain size and ensure a smooth surface for growth. Next, CH 4 was introduced into the chamber for growth. CH 4 (10 sccm) and H 2 (10 sccm) was maintained at ~750 mTorr for 30 min. Following that, the grown sheet was cooled in an atmosphere of H 2 to room temperature. The graphene on copper foil samples were coated with poly (methyl methacrylate) (PMMA) and transferred onto desired substrates. Surface preparation of single-crystal diamond, quartz and sapphire Type IIa CVD single-crystal diamonds (100) were purchased from Element Six and mechanically polished to give rms <~0.2 nm before use. Acid cleaning and hydrogen-plasma cleaning of diamond were used for all diamond samples. Metallic impurities were first dissolved in hot aqua regia (HNO 3 :HCl 1:3), followed by removing organic impurities from the diamond samples by hot ‘piranha’ solution (H 2 O 2 :H 2 SO 4 1:3) at 375 K for 1 h. H termination of diamond samples was performed by microwave hydrogen-plasma treatment using 800 W microwave power and 300 sccm of hydrogen gas flow for 15 min. Quartz (Photonics) and sapphire (MTI corporation) substrates of <0.1 nm were sequentially rinsed and sonicated in acetone, isopropyl alcohol and Nanopure water, and then dried under N 2 stream before they were used. Annealing for formation of GNB The samples were mounted on a Mo sample plate, transferred into a ultrahigh vacuum chamber with a base pressure of <10 −10 Torr. Annealing was conducted at 1,275 K for 45 min by e-beam heating (SPECS GmbH, Germany). Throughout the entire annealing process, it was ensured that the pressure did not rise beyond 10 −8 Torr. Atomic force microscopy A Dimension ICON using Nanoscope V controller (Bruker, Santa Barbra, CA) equipped with a diamond probe (DNISP; Bruker AFM Probes, Camarillo, CA) was operated in Peakforce Quantitative Nanomechanical mode for simultaneous topography imaging and Young’s modulus mapping of the graphene bubbles. In Peakforce Quantitative Nanomechanical mode, the tip is oscillated at a fixed frequency of about 2 kHz and continuously indents into the sample at a small depth of about 1–2 nm while scanning over the surface. From each indentation force curve, different physical properties such as Young’s modulus can be measured simultaneously with topography at each pixel with the same spatial and temporal resolutions ( Supplementary Fig. S5 ). Ultraviolet photoelectron emission spectroscopy The electronic structures of graphene–diamond were monitored using ultraviolet photoelectron spectroscopy. Measurements were carried out in an ultrahigh vacuum chamber (base pressure of 1 × 10 −10 Torr). The spectra were calibrated and referenced to the Fermi level gold. No charging effect was observed for all samples. During the mapping of valence band, a −5 V bias is applied to the sample to overcome the workfunction of the analyser (~4.4 eV). Raman spectroscopy Raman spectra were obtained with NEOS-SENTERRA (Bruker) AFM-raman spectrometer at room temperature, with an excitation laser source of 532 nm. The laser power was always kept <0.1 mW to prevent heating of the sample. FTIR to probe the interaction of water molecules FTIR of graphene and diamond samples were performed in the reflection mode by using an OPUS/IR PS15 spectrometer (Bruker). The sample was loaded into a high-temperature high-pressure FTIR cell evacuated to 1 × 10 −4 Torr. The spectra were the results of 32 coadded interferograms at 4 cm −1 resolution between 400 and 6,000 cm −1 with collection times of approximately 2 min. Each sample was analysed at least three times and results obtained were reproducible. MD simulations MD simulations were carried out with the reactive empirical bond-order potential potential [40] , [41] for the models containing only carbon and hydrogen atoms and with reactive force field [42] for the models containing oxygen atoms, respectively. Both methods were implemented with LAMMPS (large-scale atomic/molecular massively parallel simulation package [44] ). Periodic boundary conditions were applied in all three directions, and the MD step was 0.5 fs. Structures obtained by this procedure were visualized with the VMD package [45] . How to cite this article: Lim, CHYX et al . A hydrothermal anvil made of graphene nanobubbles on diamond. Nat. Commun. 4:1556 doi: 10.1038/ncomms2579 (2013).